Choroid plexus transcytosis and exosome shuttling deliver folate into brain parenchyma Loss of folate receptor-α function is associated with cerebral folate transport deficiency and childhood-onset neurodegeneration. To clarify the mechanism of cerebral folate transport at the blood–cerebrospinal fluid barrier, we investigate the transport of 5-methyltetrahydrofolate in polarized cells. Here we identify folate receptor-α-positive intralumenal vesicles within multivesicular bodies and demonstrate the directional cotransport of human folate receptor-α, and labelled folate from the basolateral to the apical membrane in rat choroid plexus cells. Both the apical medium of folate receptor-α-transfected rat choroid plexus cells and human cerebrospinal fluid contain folate receptor-α-positive exosomes. Loss of folate receptor-α-expressing cerebrospinal fluid exosomes correlates with severely reduced 5-methyltetrahydrofolate concentration, corroborating the importance of the folate receptor-α-mediated folate transport in the cerebrospinal fluid. Intraventricular injections of folate receptor-α-positive and -negative exosomes into mouse brains demonstrate folate receptor-α-dependent delivery of exosomes into the brain parenchyma. Our results unravel a new pathway of folate receptor-α-dependent exosome-mediated folate delivery into the brain parenchyma and opens new avenues for cerebral drug targeting. Folates are a group of essential micronutritional compounds that are found in bacteria and plants. Folic acid is a chemically synthesized, oxidized derivative that is converted to 5-methyltetrahydrofolate (5MTHF) by several enzymatic reactions. 5MTHF is the major biologically active form that functions as a cofactor in many methylation reactions. In particular, the conversion of homocysteine to methionine depends on 5MTHF. This reaction is required for the generation of S-adenosylmethionine the central methyl donor in most tissues and subcellular compartments. 5MTHF is distributed by the blood stream to all major organs where it can transverse cell membranes by at least three major transport systems [1] . The reduced folate carrier (RFC; SLC19A1) is an organic anion antiporter that exchanges 5MTHF with other inorganic or organic anions [2] . The influx Km of the RFC for 5MTHF and other reduced folates is 2–7 μM. The uptake of folates into enterocytes in the small intestine is mediated by the proton-coupled folate transporter (PCFT; SLC46A1). This transporter has a pH optimum of 5.5 and functions as proton cotransporter with a Km of about 1 μM [3] . Two glycosylphosphatidylinositol (GPI)-anchored receptors, folate receptor (FR)-α (FRα) and -β (FRβ), mediate endocytosis of folates after binding them with high affinity (Kb 1–10 nM) at neutral pH [4] , [5] . The function of the secreted FRγ and the very-low-affinity FRδ are currently not understood. In addition, several organic anion transporters (OATs) and ABC exporters (MRP1-5 and ABCG2) are capable of transporting folates with low affinity [6] , [7] . We have recently described cerebral folate transport deficiency, a childhood neurodegenerative disease that is caused by mutations in the FOLR1 gene leading to a functional loss of FRα [8] , [9] . Several other reports have confirmed the characteristics of this genetic disorder [10] , [11] . As the functional loss of FRα is associated with very low 5MTHF concentration in the cerebrospinal fluid (CSF) but normal plasma concentration of 5MTHF, and as FRα is abundantly expressed in the choroid plexus, we have hypothesized that FRα provides the major route for the blood–CSF transport of 5MTHF. In this study, we characterize the subcellular distribution of FRα and PCFT. We demonstrate that FRα mediates the transcellular 5MTHF transport into the CSF and that FRα-containing exosomes are targeted into the brain parenchyma. Localization of FRα and PCFT in the human choroid plexus To characterize the subcellular localization of FRα and PCFT in detail, an immunohistochemical analysis of sections of paraffin-embedded human choroid plexus specimens was performed. The detection with anti-human FRα antibody showed a polarized distribution of FRα, with strong staining at the apical brush border membrane and a minor FRα-signal at the basolateral membrane of the choroid plexus epithelium ( Fig. 1a ). The human PCFT was mainly detected in intracellular compartments ( Fig. 1b ). Immunofluorescence microscopy confirmed these results ( Fig. 1c ). We substantiated the reported apical localization of the RFC in the human choroids plexus ( Supplementary Fig. S1a ). The preferential apical localization of FRα seem to contradict currently held views of the role of FRα in taking up 5MTHF at the basolateral side of the choroid plexus [12] . However, these findings substantiate published results obtained in mouse and rat brain sections [13] , [14] , as well as in human tissues [15] . 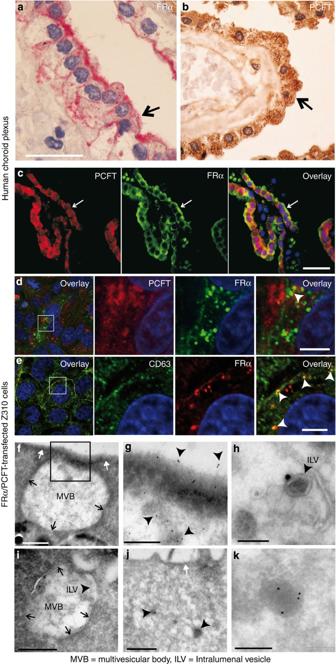Figure 1: Localization of FRα in human choroid plexus and in FRα-transfected rat choroid plexus Z310 cells. (a) Immunohistochemical staining of FRα in human choroid plexus specimen shows a predominant localization at the apical brush border membrane. A minor portion of the receptor is localized at the basolateral membrane and an intracellular punctuate staining is visible too. The arrow points to the apical membrane. Scale bar, 50 μm. (b) Immunohistochemical staining of PCFT in human choroid plexus specimen illustrates a uniformly intracellular localization with a punctate pattern. The arrow points to the apical membrane. (c) Immunofluorescence microscopy of human choroid plexus specimen demonstrates distinct distributions of PCFT (red) and FRα (green), as well as minor colocalization. Nuclei were counterstained with 4′,6-diamidino-2-phenylindole (DAPI, blue). The arrow points to the apical membrane. Scale bar, 50 μm. (d–k) Rat choroids plexus Z310 cells stably transfected with human FRα and human PCFT were fixed and prepared for immunofluorescence or electron microscopy. Confocal fluorescent microscopy of transfected Z310 cells reveals punctate PCFT (red) and FRα (green) staining (d) that colocalize only marginally. However, FRα (red) significantly colocalizes with CD63 (green), an endosomal marker that is characteristic of MVBs (e), frames indicate the magnified area. Scale bars, 5 μm. Electron microscopy after immunogold labelling of FRα demonstrates enrichment of gold particles within MVBs and close to the fusion point between MVB (black arrows) and plasma membrane (white arrows) (f). Scale bar, 500 nm. Higher magnification reveals that FRα is associated with small ILVs inside the MVB or with vesicles outside the cell (black arrowheads), (g) scale bar, 250 nm and (h) scale bar, 50 nm. Vector-tansfected Z310 cells contain similar ILV (black arrowhead) within MVBs (black arrows) but lack FRα gold staining (i), scale bar, 500 nm. PCFT staining discloses gold particles associated with medium-size electron-dense vesicles (black arrowhead) that are neither located within MVB nor fuse with the plasma membrane (white arrow), (j) scale bar, 250 nm and (k) scale bar, 100 nm. The specificity of the applied antibodies is illustrated inSupplementary Fig. S1. Figure 1: Localization of FRα in human choroid plexus and in FRα-transfected rat choroid plexus Z310 cells. ( a ) Immunohistochemical staining of FRα in human choroid plexus specimen shows a predominant localization at the apical brush border membrane. A minor portion of the receptor is localized at the basolateral membrane and an intracellular punctuate staining is visible too. The arrow points to the apical membrane. Scale bar, 50 μm. ( b ) Immunohistochemical staining of PCFT in human choroid plexus specimen illustrates a uniformly intracellular localization with a punctate pattern. The arrow points to the apical membrane. ( c ) Immunofluorescence microscopy of human choroid plexus specimen demonstrates distinct distributions of PCFT (red) and FRα (green), as well as minor colocalization. Nuclei were counterstained with 4′,6-diamidino-2-phenylindole (DAPI, blue). The arrow points to the apical membrane. Scale bar, 50 μm. ( d – k ) Rat choroids plexus Z310 cells stably transfected with human FRα and human PCFT were fixed and prepared for immunofluorescence or electron microscopy. Confocal fluorescent microscopy of transfected Z310 cells reveals punctate PCFT (red) and FRα (green) staining ( d ) that colocalize only marginally. However, FRα (red) significantly colocalizes with CD63 (green), an endosomal marker that is characteristic of MVBs ( e ), frames indicate the magnified area. Scale bars, 5 μm. Electron microscopy after immunogold labelling of FRα demonstrates enrichment of gold particles within MVBs and close to the fusion point between MVB (black arrows) and plasma membrane (white arrows) ( f ). Scale bar, 500 nm. Higher magnification reveals that FRα is associated with small ILVs inside the MVB or with vesicles outside the cell (black arrowheads), ( g ) scale bar, 250 nm and ( h ) scale bar, 50 nm. Vector-tansfected Z310 cells contain similar ILV (black arrowhead) within MVBs (black arrows) but lack FRα gold staining ( i ), scale bar, 500 nm. PCFT staining discloses gold particles associated with medium-size electron-dense vesicles (black arrowhead) that are neither located within MVB nor fuse with the plasma membrane (white arrow), ( j ) scale bar, 250 nm and ( k ) scale bar, 100 nm. The specificity of the applied antibodies is illustrated in Supplementary Fig. S1 . Full size image FRα and PCFT localize to intracellular vesicles in Z310 cells We transfected the Z310 cell line derived from immortalized rat choroid plexus cells [16] with the human FRα, PCFT, RFC or vector, respectively, and detected their expression at high resolution. Both FRα and PCFT were associated with intracellular vesicles that showed only marginal colocalization ( Fig. 1d ). FRα-positive vesicles colocalize with late endosomal markers that are characteristic for multivesicular bodies (MVBs; Fig. 1e ). Higher magnifications of MVBs by electron microscopy indicate the release of FRα-positive, intralumenal vesicles (ILVs) into the extracellular space ( Fig. 1f–h ). PCFT-positive vesicles show an electron dense lumen and are not associated with MVBs ( Fig. 1j ). Basolateral to apical transport of FRα in polarized cells We studied the transport of labelled folates in cultures of polarized cells and used the rat choroid plexus Z310 cells as a model system. Filter-grown Z310 cells, stably expressing FRα, were incubated with fluorescein isothiocyanate (FITC)-labelled folic acid (FA-FITC). Anti-FRα antibody was added to the basolateral medium of the cells. Imaging of cells at various time points (0, 60 and 120 min) revealed FRα redistribution from the basolateral to the apical membrane ( Fig. 2a–c ). In contrast, after apical labelling no redistribution of FRα but a loss of fluorescence signal was observed, indicating unidirectional basolateral to apical transcytosis of FRα and release of FRα from the apical membrane ( Fig. 2d ). 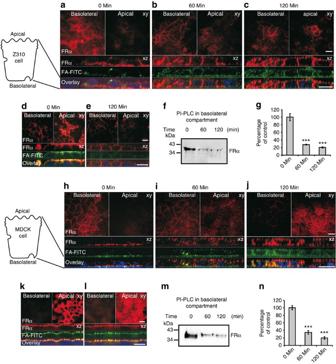Figure 2: Transcytosis of FRα in the polarized cell lines Z310 and MDCK. (a–c) FRα-expressing Z310 cells were incubated on ice for 15 min with FA-FITC, together with anti-human FRα antibody added to the basolateral chamber of the transwell plate. Filters were fixed immediately (a) or were shifted to 37 °C for 60 min (b) or 120 min (c), and were analysed by confocal microscopy;xyandxzimages reveal that the antibody (red) and FA-FITC (green) initially bind to FRα at the basolateral surface of the cells (a) whereas after 60 min and 120 min the antibody together with FA-FITC were transported to the apical surface of the cells (b,c). When FA-FITC and antibody were added to the apical chamber of the transwell plate, no transcytosis to the basolateral membrane was observed after 120 min (d). Both FA-FITC and antibody disappeared at the apical surface, suggesting a release of FRα from the apical membrane (e). (f) When PI-PLC was added for 60 min or 120 min to the basolateral surface of FRα-expressing Z310 cells, the amount of apically sorted FRα diminished over time as displayed by western blotting and quantified by densitometry (g). Values are means±s.e.m. of three independent experiments. Statistical analysis was done by Student’st-test (***P<0.001). (h–j) FRα-expressing MDCK cells were incubated with FA-FITC together with anti-human FRα antibody as described for the Z310 cells. Filters were fixed immediately (h) or were shifted to 37 °C for 60 min (i) or 120 min (j), and were analysed by confocal microscopy. Antibody (red) and FA-FITC (green) initially bind to FRα at the basolateral surface of the cells (h), whereas after 60 min (i) and 120 min (j) the antibody and FA-FITC become redistributed to the apical surface of the cells. When FA-FITC and antibody were added to the apical chamber (k), no transcytosis to the basolateral membrane was observed after 120 min (l). In contrast to Z310 cells, no decrease of the apical fluorescent staining was observed. Scale bar fora–eandh–l, 10 μm. When PI-PLC was added for 60 min or 120 min to the basolateral surface of FRα-expressing MDCK cells, apically sorted FRα diminished over time as displayed by western blotting (m) and quantified by densitometry (n). Values are means±s.e.m. of three independent experiments (***P<0.001; Student’st-test). Full-scan images are displayed inSupplementary Fig. S6. Figure 2: Transcytosis of FRα in the polarized cell lines Z310 and MDCK. ( a – c ) FRα-expressing Z310 cells were incubated on ice for 15 min with FA-FITC, together with anti-human FRα antibody added to the basolateral chamber of the transwell plate. Filters were fixed immediately ( a ) or were shifted to 37 °C for 60 min ( b ) or 120 min ( c ), and were analysed by confocal microscopy; xy and xz images reveal that the antibody (red) and FA-FITC (green) initially bind to FRα at the basolateral surface of the cells ( a ) whereas after 60 min and 120 min the antibody together with FA-FITC were transported to the apical surface of the cells ( b , c ). When FA-FITC and antibody were added to the apical chamber of the transwell plate, no transcytosis to the basolateral membrane was observed after 120 min ( d ). Both FA-FITC and antibody disappeared at the apical surface, suggesting a release of FRα from the apical membrane ( e ). ( f ) When PI-PLC was added for 60 min or 120 min to the basolateral surface of FRα-expressing Z310 cells, the amount of apically sorted FRα diminished over time as displayed by western blotting and quantified by densitometry ( g ). Values are means±s.e.m. of three independent experiments. Statistical analysis was done by Student’s t -test (*** P <0.001). ( h – j ) FRα-expressing MDCK cells were incubated with FA-FITC together with anti-human FRα antibody as described for the Z310 cells. Filters were fixed immediately ( h ) or were shifted to 37 °C for 60 min ( i ) or 120 min ( j ), and were analysed by confocal microscopy. Antibody (red) and FA-FITC (green) initially bind to FRα at the basolateral surface of the cells ( h ), whereas after 60 min ( i ) and 120 min ( j ) the antibody and FA-FITC become redistributed to the apical surface of the cells. When FA-FITC and antibody were added to the apical chamber ( k ), no transcytosis to the basolateral membrane was observed after 120 min ( l ). In contrast to Z310 cells, no decrease of the apical fluorescent staining was observed. Scale bar for a – e and h – l , 10 μm. When PI-PLC was added for 60 min or 120 min to the basolateral surface of FRα-expressing MDCK cells, apically sorted FRα diminished over time as displayed by western blotting ( m ) and quantified by densitometry ( n ). Values are means±s.e.m. of three independent experiments (*** P <0.001; Student’s t -test). Full-scan images are displayed in Supplementary Fig. S6 . Full size image To confirm the basolateral origin of the apically detected FRα protein, we removed FRα by the addition of phosphatidylinositol-specific phospholipase C (PI-PLC) to the basolateral medium. After incubation for 0, 60 and 120 min, FRα was released from the apical membrane by the addition of PI-PLC to the apical medium. Western blot analysis revealed a gradual reduction of FRα signal by maximal 76% after 120 min incubation ( Fig. 2f ). This basolateral to apical cotransport of FRα, together with FITC-labelled folic acid, could be replicated in experiments with Madin–Darby canine kidney (MDCK) cells that were stably transfected with FRα ( Fig. 2h–n ). However, in case of MDCK cells no significant reduction in apical fluorescence was observed after apical labelling and 120 min incubation ( Fig. 2k ). This suggests that in contrast to Z310 cells, MDCK cells do not release FRα from the apical surface. We additionally analysed the distribution of FRα in HepG2 cells stably transfected with the human FOLR1 cDNA. FRα accumulated at the apical bile canalicular membrane and was less intensively expressed at the basolateral membrane ( Supplementary Fig. S2a ). Blocking of vesicular membrane fusion by preincubation of HepG2 cells with N-ethylmaleimide resulted in reduced basolateral FRα staining ( Supplementary Fig. S2b ). Preincubation with brefeldin A to block Golgi-to-cell surface traffic resulted in preferential basolateral FRα staining, indicating a disturbed FRα trafficking even though FRα internalization was preserved ( Supplementary Fig. S2c ). These data support the notion of a vesicular transport of FRα from the basolateral to the apical membrane in polarized cells. Exosomal FRα expression correlates with 5MTHF in human CSF To understand the mechanism of FRα shedding into the CSF, we fractionated human CSF by sequential centrifugation with increasing centrifugal forces. Surprisingly, FRα was enriched in the P100 (100,000 g ) fraction containing small vesicles with a diameter of 40–100 nm and colocalizing with exosomal markers such as flotillin-2 (Flot-2) and Alix ( Fig. 3a–d ). Immunoelectron microscopy revealed the presence of FRα at the surface of exosomes, and two-colour stimulated emission depletion (STED) microscopy [17] , [18] confirmed the vesicle-specific colocalization of FRα with the exosomal marker Alix ( Fig. 3c ). From the same STED data, the exact vesicle size could be assessed ( Fig. 3e ) and a quantitative colocalization of FRα with Alix was determined to be in the range of 36±8%. 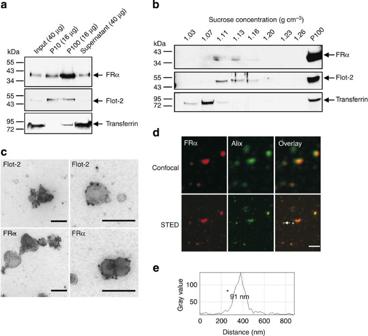Figure 3: Identification and characterization of FRα-positive exosomes in specimen of human CSF. (a) Sequential centrifugation steps were conducted with human CSF specimen and the resulting pellets were analysed by western blotting. P10 refers to the pellet from 10,000gcentrifugation step; P100 refers to the pellet from 100,000gcentrifugation step. The input and the remaining supernatants after the 100,000gcentrifugation were concentrated 20-fold prior loading on the gel. FRα and the exosomal marker Flot-2 are enriched in P100, whereas transferrin remains mainly in the supernatant. Full-scan images are displayed inSupplementary Fig. S6. (b) A 100,000gpellet was loaded on top of a discontinuous sucrose density gradient and ultracentrifuged for 16 h. The fractions were then analysed by western blotting. FRα is enriched in the same fractions as Flot-2. Full-scan images are displayed inSupplementary Fig. S6. (c) For electron microscopy, a 100,000gpellet was negatively stained with uranyl acetate and immunolabelled with antibodies against FRα or Flot-2. The pellet contains mainly small membrane vesicles with a diameter of about 40–100 nm, with the typical cup-shaped morphology of exosomes, that are positive for FRα and Flot-2. Scale bars, 200 nm. (d) High-resolution imaging of the 100,000gpellet and colocalization analysis of FRα and the exosomal marker Alix by two-colour STED microscopy. Although standard confocal microscopy fails to display the details, STED microscopy reveals the typical size of exosomes and analysis of the images demonstrates a colocalization of FRα with Alix of 36%±8% (data calculated with the NIH Image J software). Scale bar, 1 μm. (e) STED microscopy allows exact size determination of the vesicles positive for FRα and Alix (arrowhead ind). Figure 3: Identification and characterization of FRα-positive exosomes in specimen of human CSF. ( a ) Sequential centrifugation steps were conducted with human CSF specimen and the resulting pellets were analysed by western blotting. P10 refers to the pellet from 10,000 g centrifugation step; P100 refers to the pellet from 100,000 g centrifugation step. The input and the remaining supernatants after the 100,000 g centrifugation were concentrated 20-fold prior loading on the gel. FRα and the exosomal marker Flot-2 are enriched in P100, whereas transferrin remains mainly in the supernatant. Full-scan images are displayed in Supplementary Fig. S6 . ( b ) A 100,000 g pellet was loaded on top of a discontinuous sucrose density gradient and ultracentrifuged for 16 h. The fractions were then analysed by western blotting. FRα is enriched in the same fractions as Flot-2. Full-scan images are displayed in Supplementary Fig. S6 . ( c ) For electron microscopy, a 100,000 g pellet was negatively stained with uranyl acetate and immunolabelled with antibodies against FRα or Flot-2. The pellet contains mainly small membrane vesicles with a diameter of about 40–100 nm, with the typical cup-shaped morphology of exosomes, that are positive for FRα and Flot-2. Scale bars, 200 nm. ( d ) High-resolution imaging of the 100,000 g pellet and colocalization analysis of FRα and the exosomal marker Alix by two-colour STED microscopy. Although standard confocal microscopy fails to display the details, STED microscopy reveals the typical size of exosomes and analysis of the images demonstrates a colocalization of FRα with Alix of 36%±8% (data calculated with the NIH Image J software). Scale bar, 1 μm. ( e ) STED microscopy allows exact size determination of the vesicles positive for FRα and Alix (arrowhead in d ). Full size image The importance of FRα release into the CSF was further investigated by western blotting with human CSF from both healthy individuals and patients with cerebral folate transport deficiency. FRα could be detected in CSF of controls but was absent from patients that carry pathogenic FOLR1 mutations ( Fig. 4a ). As we have shown intracellular expression of the FRα missense mutants p.C65W, p.C169Y and p.N222S [9] their absence in CSF indicate a disturbed export of these FRα mutants. The absence of FRα was associated with a severely diminished concentration of 5MTHF in the CSF, equal to or below 5 nM in untreated patients (normal range 40–120 nM). To test whether low CSF concentrations of 5MTHF are correlated with low or absent CSF detection of FRα in other disorders, we investigated patients with Kearns–Sayre syndrome (KSS), a mitochondrial disorder with disturbed blood–CSF transport of 5MTHF due to failure of the choroid plexus [19] , [20] . CSF samples obtained at different time points but from the same patient were compared ( Fig. 4b ). The sample with the slightly reduced 5MTHF concentration in the CSF of 39.4 nM showed a decreased but detectable FRα signal. In contrast, CSF FRα was hardly detectable in the sample where the CSF 5MTHF was below 5 nM. The CSF samples of eight additional patients with KSS showed a similar corrleation between 5MTHF concentration and level of FRα expression( Fig. 4c ). These findings suggest a link between CSF 5MTHF and CSF FRα, and indicate a crucial role of the choroid plexus in the export and maintenance of 5MTHF and FRα in the CSF. 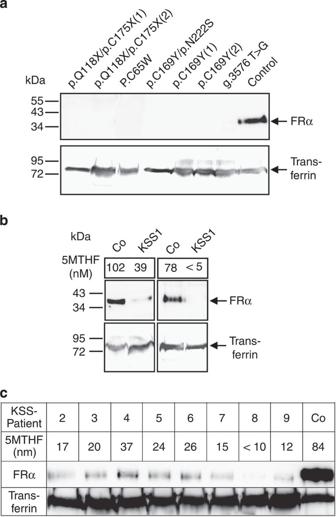Figure 4: Detection of FRα in CSF by western blotting. (a) CSF of patients with cerebral folate transport deficiency and controls, respectively, were concentrated tenfold using ‘Amicon Centrifugal Filter Devices’. Thirty micrograms of protein per lane were subjected to SDS–PAGE and western blotting. FRα is absent in the CSF of patients with cerebral folate transport deficiency while it can be clearly detected in the control samples (only one of five different shown). The patients carry the following mutations in theFOLR1gene: the compound heterozygous mutations p.Q118X/p.C175X and p.C169Y/p.N222S, the homozygous mutations p.C65W and p.169Y and the homozygous splice site mutation g.3576T>G. Full-scan images are displayed inSupplementary Fig. S6. The amount of FRα in the CSF correlates with the concentration of 5MTHF in the CSF (b,c). Two CSF samples from one patient that was diagnosed with KSS, a mitochondrial disorder that is associated with reduced concentration of 5MTHF in the CSF, were compared. The sample with 5MTHF concentration of 39.4 nmol l−1(reference value: 40–120 nmol l−1) showed a diminished amount of FRα in the CSF, whereas in the second sample the 5MTHF concentration in the CSF was below 5 nmol l−1and FRα was not detectable (b). CSF samples (100 μg each) from eight additional patients with genetically confirmed KSS were analysed by western blotting. The intensity of the FRα signal roughly correlated with the 5MTHF concentration in the CSF (c). Transferrin served as loading control. Full-scan images are displayed inSupplementary Fig. S6. Figure 4: Detection of FRα in CSF by western blotting. ( a ) CSF of patients with cerebral folate transport deficiency and controls, respectively, were concentrated tenfold using ‘Amicon Centrifugal Filter Devices’. Thirty micrograms of protein per lane were subjected to SDS–PAGE and western blotting. FRα is absent in the CSF of patients with cerebral folate transport deficiency while it can be clearly detected in the control samples (only one of five different shown). The patients carry the following mutations in the FOLR1 gene: the compound heterozygous mutations p.Q118X/p.C175X and p.C169Y/p.N222S, the homozygous mutations p.C65W and p.169Y and the homozygous splice site mutation g.3576T>G. Full-scan images are displayed in Supplementary Fig. S6 . The amount of FRα in the CSF correlates with the concentration of 5MTHF in the CSF ( b , c ). Two CSF samples from one patient that was diagnosed with KSS, a mitochondrial disorder that is associated with reduced concentration of 5MTHF in the CSF, were compared. The sample with 5MTHF concentration of 39.4 nmol l −1 (reference value: 40–120 nmol l −1 ) showed a diminished amount of FRα in the CSF, whereas in the second sample the 5MTHF concentration in the CSF was below 5 nmol l −1 and FRα was not detectable ( b ). CSF samples (100 μg each) from eight additional patients with genetically confirmed KSS were analysed by western blotting. The intensity of the FRα signal roughly correlated with the 5MTHF concentration in the CSF ( c ). Transferrin served as loading control. Full-scan images are displayed in Supplementary Fig. S6 . Full size image 5MTHF transport across the choroid plexus is mediated by FRα To reconcile our experimental data from polarized cells with the presence of FRα-expressing exosomes in the CSF, we studied the transcellular transport of 5MTHF across the choroid plexus. For this purpose, we investigated the directed movements of radioactively labelled 5MTHF across Z310 cells as well as across primary porcine choroid plexus epithelial cells (PCPECs). FRα-transfected or vector control-transfected Z310 cells were grown in a two chamber transwell system, and [ 3 H]5MTHF was either given into the basolateral or apical compartment. In short-term experiments over 3 h [ 3 H]5MTHF was merely taken up by FRα-transfected Z310 cells from both compartments, and vectorial transport could only be detected when PI-PLC was added to the apical compartment ( Supplementary Fig. S3 ). For extended studies, the radioactive medium was replaced with fresh medium after 1 h incubation to prevent transepithelial diffusion of [ 3 H]5MTHF. During the extended 48 h incubation, [ 3 H]5MTHF emerged in the apical compartment of FRα-transfected but not vector-transfected cells ( Fig. 5a ). Moreover, apical shedding of [ 3 H]5MTHF was increased upon addition of either monensin (70% increase) or transferrin (36% increase). The monensin- or transferrin-dependent increase in apical release occurred at the expense of the intracellular [ 3 H]5MTHF uptake. Whether Z310 cells were loaded with [ 3 H]MTHF from the apical or basolateral site did not significantly alter the rate of apical shedding, but no significant basolateral release of [ 3 H]5MTHF could be detected under any condition. As monensin and transferrin induce exosome release from cells [21] , these data further suggest an exosomal type of FRα-mediated transport of 5MTHF into the apical compartment. 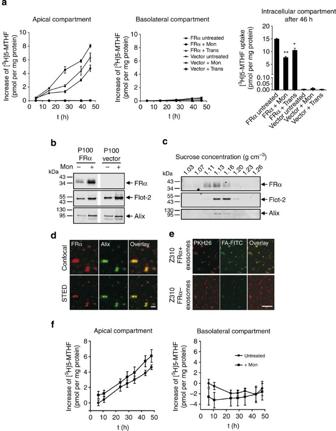Figure 5: FRα-mediated transport of 5MTHF in Z310 cells is stimulated by monensin and transferrin. (a) Filter-grown Z310 cells stably transfected with FRα or vector were loaded with [3H]5MTHF for 1 h. After three washing steps, cells were incubated with fresh RPMI medium containing either 7 μM monensin (Mon), 0.5 mg ml−1rat transferrin (Trans) or no supplementation. Samples from the apical and basolateral compartment were removed at the indicated time points. Subsequently, cells were lysed and radioactivity was measured in medium samples and cell lysates. Data are means±s.e.m. of three independent experiments (**P<0.01; *P<0.05; Student’st-test). (b) Z310 cells stably transfected with FRα or vector were treated with 7 μM monensin for 22 h. The medium was collected and subjected to ultracentrifugation for exosome purification. The P100 pellets were analysed by western blotting and probed with antibodies against FRα, Flot-2 and Alix. Full-scan images are displayed inSupplementary Fig. S6. (c) To further characterize the vesicles derived from Z310 cells, the 100,000gpellet from monensin-treated Z310 cells stably expressing FRα was subjected to sucrose gradient ultracentrifugation. FRα is mainly enriched in the fractions that contained Flot-2 and Alix. Full-scan images are displayed inSupplementary Fig. S6. (d) Two-colour STED microscopy of exosomes purified from Z310 cells stably expressing FRα demonstrates a colocalization of FRα with Alix of 63%±13% (data calculated with the NIH Image J software). Scale bar, 1 μm. (e) Exosomes purified from either FRα-transfected or vector-transfected Z310 cells were stained with the dye PKH26 before they were incubated with FITC-FA for 1 h at RT. Only FRα-positive exosomes colocalize with FITC-FA and thus bind folate. Scale bar, 20 μm. (f) Apical transport of 5MTHF in primary PCPECs. Filter-grown PCPECs were loaded with 25 nM [3H]5MTHF for 24 h. Cells were then incubated with 7 μM monensin or left untreated. Radioactivity from apical medium samples was measured at the indicated time points. The increase of the apical [3H]5MTHF concentration was further enhanced by incubating the cells with monensin. Data are means±s.e.m. of two independent experiments, each done in triplicate. Figure 5: FRα-mediated transport of 5MTHF in Z310 cells is stimulated by monensin and transferrin. ( a ) Filter-grown Z310 cells stably transfected with FRα or vector were loaded with [ 3 H]5MTHF for 1 h. After three washing steps, cells were incubated with fresh RPMI medium containing either 7 μM monensin (Mon), 0.5 mg ml −1 rat transferrin (Trans) or no supplementation. Samples from the apical and basolateral compartment were removed at the indicated time points. Subsequently, cells were lysed and radioactivity was measured in medium samples and cell lysates. Data are means±s.e.m. of three independent experiments (** P <0.01; * P <0.05; Student’s t -test). ( b ) Z310 cells stably transfected with FRα or vector were treated with 7 μM monensin for 22 h. The medium was collected and subjected to ultracentrifugation for exosome purification. The P100 pellets were analysed by western blotting and probed with antibodies against FRα, Flot-2 and Alix. Full-scan images are displayed in Supplementary Fig. S6 . ( c ) To further characterize the vesicles derived from Z310 cells, the 100,000 g pellet from monensin-treated Z310 cells stably expressing FRα was subjected to sucrose gradient ultracentrifugation. FRα is mainly enriched in the fractions that contained Flot-2 and Alix. Full-scan images are displayed in Supplementary Fig. S6 . ( d ) Two-colour STED microscopy of exosomes purified from Z310 cells stably expressing FRα demonstrates a colocalization of FRα with Alix of 63%±13% (data calculated with the NIH Image J software). Scale bar, 1 μm. ( e ) Exosomes purified from either FRα-transfected or vector-transfected Z310 cells were stained with the dye PKH26 before they were incubated with FITC-FA for 1 h at RT. Only FRα-positive exosomes colocalize with FITC-FA and thus bind folate. Scale bar, 20 μm. ( f ) Apical transport of 5MTHF in primary PCPECs. Filter-grown PCPECs were loaded with 25 nM [ 3 H]5MTHF for 24 h. Cells were then incubated with 7 μM monensin or left untreated. Radioactivity from apical medium samples was measured at the indicated time points. The increase of the apical [ 3 H]5MTHF concentration was further enhanced by incubating the cells with monensin. Data are means±s.e.m. of two independent experiments, each done in triplicate. Full size image FRα released from choroids plexus cells is bound to exosomes The vesicular nature of the directed FRα-dependent transport was confirmed by fractionation of the apical cell culture supernatant from FRα-transfected Z310 cells. FRα was enriched in the P100 (100,000 g pellet) fraction and was copurified with the exosomal markers Flot-2 and Alix ( Fig. 5b ). The monensin-induced increase in FRα signal was proportional to the increase in Flot-2 and Alix release. Flot-2 and Alix release was also induced by monensin in vector-transfected cells in the absence of FRα. The vesicle-containing P100 fraction of FRα-transfected and monensin-treated Z310 cells were subjected to sucrose gradient ultracentrifugation. Very similar to human CSF ( Fig. 3b ), FRα was mainly recovered from fractions possessing the characteristic density of exosomes (between 1.11 and 1.16 g cm −3 ) and containing the exosomal markers Flot-2 and Alix ( Fig. 5c ). About 80% of the total FRα in the apical supernatant was present in the P100 fraction and this corresponds to the proportion of [ 3 H]5MTHF that was recovered in the P100 fraction ( Supplementary Table S1 ). The isolated vesicles showed the typical size of exosomes and could be costained for FRα and Alix in two-colour STED microscopy ( Fig. 5d ). Quantitative analysis revealed a colocalization of 63±8% of FRα and Alix. Incubation of PKH26-labelled FRα-positive and FRα-negative exosomes with FITC-labelled folic acid revealed specific colocalization of FITC-FA with FRα-positive exosomes ( Fig. 5e ). These data demonstrate that exosomes derived from FRα-expressing Z310 cells bind folates and share major characteristics with exosomes derived from human CSF. The fact that quantitative analysis of STED images achieved a higher percentage of FRα colocalization with the exosomal marker Alix can be explained by the overexpression of FRα in Z310 cells. We also compared the protein composition of exosome preparations derived from Z310 cells with the one purified from human CSF by mass spectrometry ( Table 1 ). Both preparations contained 84–88% commonly accepted exosomal markers [22] and showed an overall similar protein profile. Table 1 Mass spectrometry analysis of exosomes purified from human CSF or from the supernatant of transfected rat choroid plexus Z310 cells. Full size table To validate our findings in Z310 cells, we studied the directional 5MTHF transport in primary PCPECs. Filter-grown PCPECs were loaded with 25 nM [ 3 H]5MTHF for 24 h. Subsequently, medium was changed and cells were treated with 7 μM monensin or left untreated. A significant increase of radioactivity could only be observed in the apical compartment ( Fig. 5f ). Treatment of cells with monensin further enhanced the apical accumulation of [ 3 H]5MTHF by 33%. The rate of transport into the apical compartment corresponded to the rate obtained for FRα-transfected Z310 cells. Equivalent to Z310 cells, about 70% of the [ 3 H]5MTHF was recovered in the P100 fraction and no significant [ 3 H]5MTHF release was detected in the basolateral compartment. The supernatant of FRα-transfected MDCK cells (see Fig. 2h–n ) were also fractionated but did not reveal any significant amount of vesicles in the P100 fraction and did not contain detectable exosomal markers or FRα. Correspondingly, no exosomal release of 5MTHF at the apical plasma membrane could be measured. We performed additional experiments to evaluate FRα-independent transport processes in Z310 cells at physiological 5MTHF concentration (12.5 nM). A couple of organic anion transporters are known to be expressed in Z310 cells [23] . Contribution of Oat1, Oat3, Oatp2, Oatp3, Mrp1, Mrp4, p-glycoprotein (Mdr1) and RFC to 5MTHF uptake into FRα-transfected Z310 cells was assessed by the incubation of cells with the following inhibitors of these transporters: taurocholate, methotrexate (MTX), p-aminohippuric acid, probenecid and digoxin. As illustrated in Supplementary Fig. S4 , none of the inhibitors reduced the uptake of [ 3 H]5MTHF with the exception of MTX. However, at the 10 μM concentration of MTX this antifolate is known to competitively block binding of 5MTHF to FRα as well. FRα-associated 5MTHF is transported across the choroid plexus The contribution of the PCFT and the RFC to FRα-mediated 5MTHF transport by Z310 cells was further studied by stable cotransfection of FRα with PCFT or RFC, or a combination of both. Free (=cytosolic) and endosomal (=vesicular) 5MTHF was compared between FRα-transfected and FRα- plus PCFT-transfected Z310 cells ( Supplementary Fig. S5a ). Although the amount of cytosolic 5MTHF was slightly higher in FRα/PCFT-double-transfected Z310 cells, there was no significant differences in the endosomal 5MTHF fraction. The transfection of FRα increased the 5MTHF uptake 248-fold when compared with the vector-transfected control cells. Additional transfection with PCFT or RFC, or the combination of both, did not significantly alter 5MTHF uptake into Z310 cells when compared with the control cells ( Supplementary Fig. S4b ). Further, knocking down endogenously expressed PCFT and RFC by specific short interfering RNAs did not alter the FRα-mediated 5MTHF transport ( Supplementary Fig S4c,d ). These data indicate that at least at the physiological 5MTHF concentrations in plasma (4–20 nM), the major proportion of 5MTHF that is captured by FRα at the basolateral site of the choroid plexus, is transcytosed and released from the apical border of the choroid plexus. FRα-positive exosomes penetrate into brain parenchyma in vivo We have unexpectedly discovered the release of FRα as exosomal cargo into the CSF. To further understand the biological function of this transport mechanism, we injected exosomes derived from FRα-transfected or vector-transfected Z310 cells into the lateral ventricle of C57BL/6 mice. Purified exosomes were labelled with the dye PKH26 before they were applied via stereotactically implanted intraventricular cannulas. Four hours post injection, the mice were killed and their brains immediately frozen. Immunohistochemistry of the mouse brain sections revealed that FRα-positive exosomes penetrated into the brain parenchyma distal from the injection site and colocalized with glial fibrillary acidic protein (GFAP)-positive astrocytes as well as NeuN-positive neurons ( Fig. 6a ). In contrast, FRα-negative exosomes were mainly detected close to the periventricular ependyma. No parenchymal staining was observed after injection of 100 nM FA-FITC into the mouse brain ventricles. 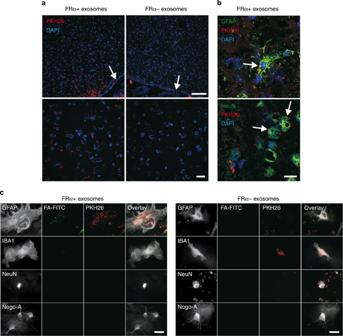Figure 6: FRα-expressing exosomes penetrate into the brain parenchymain vivoand are internalized by astrocytesin vitro. (a) Exosomes were purified from the cell culture supernatant of transfected Z310 cells and labelled with the dye PKH26 (red). Ten microlitres of the exosome solutions were then injected in mice with surgical implanted intraventricular cannulas 4 h before the mice were killed. Immunofluorescent staining of the mouse brain sections shows that exosomes derived from FRα-transfected Z310 cells (FRα+) cross the ependymal cell layer and are distributed deeply in the brain parenchyma distal from the injection site. In contrast, exosomes derived from vector-transfected cells (FRα-) cannot penetrate the parenchyma but are retained at the ependyma. Nuclei were counterstained with DAPI (blue). Upper scale bar, 100 μm, lower scale bar, 20 μm. (b) Immunostaining of the mouse brain sections with antibodies against GFAP and NeuN reveal that exosomes (red) derived from FRα-transfected Z310 cells colocalize with GFAP-positive astrocytes and NeuN-positive neurons. Nuclei were counterstained with DAPI (blue). Scale bar, 10 μm. (c) Purified exosomes from Z310 cells were labelled with the dye PKH26 (red), incubated with FA-FITC (green) and added to primary mixed cortical cultures on daysin vitro(DIV) 7, consisting of mouse oligodendrocytes, astrocytes, cortical neurons and microglia. After incubation with exosomes for 2 h at 37 °C, the cells were fixed and analysed by immunofluorescence microscopy. Oligodendrocytes, astrocytes, neurons and microglia were recognized by antibodies against Nogo-A, GFAP, Iba1 and NeuN. The primary antibodies were recognized with secondary biotin-conjugated antibodies and subsequently labelled with streptavidin-coupled Pacific blue (shown in grey for better visualisation). FRα-containing exosomes (FRα+) are selectively taken up by GFAP-positive astrocytes. Partial colocalization of FA-FITC and PKH26 is also observed in these cells. Exosomes purified from the culture medium of vector-transfected Z310 cells (FRα-) are not taken up by astrocytes but are internalized by Iba1-positive microglia. Note that none of the cell types was found to internalize free FA-FITC. Scale bar: 20 μm. Figure 6: FRα-expressing exosomes penetrate into the brain parenchyma in vivo and are internalized by astrocytes in vitro . ( a ) Exosomes were purified from the cell culture supernatant of transfected Z310 cells and labelled with the dye PKH26 (red). Ten microlitres of the exosome solutions were then injected in mice with surgical implanted intraventricular cannulas 4 h before the mice were killed. Immunofluorescent staining of the mouse brain sections shows that exosomes derived from FRα-transfected Z310 cells (FRα+) cross the ependymal cell layer and are distributed deeply in the brain parenchyma distal from the injection site. In contrast, exosomes derived from vector-transfected cells (FRα-) cannot penetrate the parenchyma but are retained at the ependyma. Nuclei were counterstained with DAPI (blue). Upper scale bar, 100 μm, lower scale bar, 20 μm. ( b ) Immunostaining of the mouse brain sections with antibodies against GFAP and NeuN reveal that exosomes (red) derived from FRα-transfected Z310 cells colocalize with GFAP-positive astrocytes and NeuN-positive neurons. Nuclei were counterstained with DAPI (blue). Scale bar, 10 μm. ( c ) Purified exosomes from Z310 cells were labelled with the dye PKH26 (red), incubated with FA-FITC (green) and added to primary mixed cortical cultures on days in vitro (DIV) 7, consisting of mouse oligodendrocytes, astrocytes, cortical neurons and microglia. After incubation with exosomes for 2 h at 37 °C, the cells were fixed and analysed by immunofluorescence microscopy. Oligodendrocytes, astrocytes, neurons and microglia were recognized by antibodies against Nogo-A, GFAP, Iba1 and NeuN. The primary antibodies were recognized with secondary biotin-conjugated antibodies and subsequently labelled with streptavidin-coupled Pacific blue (shown in grey for better visualisation). FRα-containing exosomes (FRα+) are selectively taken up by GFAP-positive astrocytes. Partial colocalization of FA-FITC and PKH26 is also observed in these cells. Exosomes purified from the culture medium of vector-transfected Z310 cells (FRα-) are not taken up by astrocytes but are internalized by Iba1-positive microglia. Note that none of the cell types was found to internalize free FA-FITC. Scale bar: 20 μm. Full size image FRα-positive exosomes are internalized by astrocytes in vitro To further confirm these in vivo findings, we incubated primary mixed cortical cultures obtained from neonatal mice with either PKH26-labelled exosomes, with FA-FITC or a combination of both. After incubating the cells for 2 h at 37 °C, cells were fixed and analysed by immunofluorescence microscopy. FRα-positive exosomes were selectively taken up by GFAP-positive astrocytes but no significant colocalization was obtained with cells stained with markers for microglia, neurons and oligodendrocytes ( Fig. 6c ). FRα-negative exosomes did not colocalize with astrocytes but were internalized by Iba1-positive microglia. FA-FITC was also delivered to astrocytes when combined with FRα-positive exosomes. However, none of the cell types internalized 100 nM of free FA-FITC. Several characteristics of FRα argue for its pivotal role in the 5MTHF transport across the blood–CSF barrier. Within the brain FRα is almost selectively expressed in the choroid plexus and its high binding affinity for folates (Kb 1–10 nM) perfectly matches the physiological 5MTHF concentration in human plasma (4–20 nM). Further, a hereditary FRα defect causes extremely low 5MTHF concentrations in the CSF (equal or below 5 nM) and results in a childhood onset neurodegenerative disease [8] , [9] . In addition, the occurrence of FRα autoantibodies in plasma is associated with low 5MTHF concentration in the CSF as well as with a similar neurodegenerative disease [24] . Our experiments with various polarized cells (MDCK, HepG2, Z310 cells) demonstrate a basolateral to apical sorting of FRα that provides for receptor-mediated endocytosis and transcytosis of folates ( Fig. 2 and Supplementary Fig. S2 ). These findings indicate that the GPI-anchored FRα promote a vesicular transport of 5MTHF across the choroid plexus. GPI-anchored proteins are known to be associated with specific subcellular compartments. They enter the endosomal compartment by a clathrin-independent pathway to form tubular early endocytic compartments called GPI-anchored protein-enriched endosomal compartments [25] , [26] . Our data indicate FRα translocation to maturated endosomes that are named MVBs and that contain ILVs. MVBs are known to be sites for intracellular sorting of proteins between recycling, degradation and secretion pathways [27] . We have provided several lines of evidence that in choroid plexus cells FRα-containing MVBs fuse with the apical membrane and secrete their ILVs as exosomes ( Fig. 1e–h , Fig. 7 ). We further suggest that FRα recycles between the apical membrane and the late endosomal compartment, and thus offers 5MTHF uptake from the CSF as well. The absence of effect in folate binding and transport after transfection of human PCFT and human RFC or after short interfering RNA suppression of endogenous rat PCFT and rat RFC indicates the essential role of FRα-mediated transport of 5MTHF at its physiological concentration ( Supplementary Fig. S5b–d ). Further, the pharmacological inhibition of various folate transporters did not alter folate binding to Z310 choroid plexus cells ( Supplementary Fig. S4 ). These results are consistent with recent studies on primary rat choroid plexus epithelial cells that show two separate folate uptake mechanisms [28] . One FRα-dependent process mediates efficient uptake of 5MTHF at low extracellular folate concentrations. The other uptake mechanism is independent of FRα but likely depends on organic transporters, such as the RFC, and accounts for folate uptake at higher concentrations. It is possible that in case of abundant folate supply 5MTHF may follow other routes of internalization and transport in the choroid plexus. However, it is likely that any free 5MTHF released into the CSF will be picked up by membrane-attached FRα either present on exosomes or on the apical surface of the choroid plexus. As about 36% of all human CSF exosomes contain FRα ( Fig. 3d ) and as the brain FRα exclusively origins from the choroid plexus [8] , we consider the human choroid plexus as a major source of CSF exosomes. 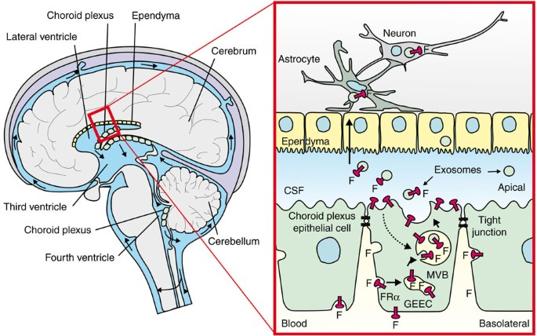Figure 7: Suggested model of human cerebral folate transport. Schematic drawing of the brain including the cerebrospinal fluid circulation. The rectangle indicates the magnified area containing the choroid plexus and the ependyma. At physiological plasma concentrations (6–40 nM) 5MTHF (F) is primarily taken up by FRα at the basolateral membrane of the human choroid plexus. The 5MTHF-FRα complex is internalized by receptor-mediated endocytosis, translocated into GPI-anchored protein-enriched early endosomal compartments (GEECs) and further transferred to MVBs. MVBs are late endosomal compartments localized in the endocytic route. A minor proportion of internalized 5MTHF is translocated to PCFT-positive vesicles and transported into the cytoplasma. ILVs of MVBs containing FRα are generated by inward budding of the limiting membrane. These ILVs are released as exosomes into the CSF after fusion of the MVB with the apical cell membrane. Fusion of the limiting membrane of MVBs with the apical membrane explains the presence of FRα molecules on the apical surface of the choroid plexus cells too. FRα-containing exosomes circulate in the CSF, cross the ependymal cell layer and are distributed in the brain parenchyma. FRα-positive exosomes might initially be taken up by astrocytes and from these further delivered to neurons. FRα-negative exosomes hardly cross the ependymal cell layer and are targeted to other brain cells, such as microglia. At higher than normal plasma concentrations of 5MTHF (>100 nM) alternative mechanisms of uptake and transport may provide for transcellular 5MTHF delivery across the choroid plexus. Figure 7: Suggested model of human cerebral folate transport. Schematic drawing of the brain including the cerebrospinal fluid circulation. The rectangle indicates the magnified area containing the choroid plexus and the ependyma. At physiological plasma concentrations (6–40 nM) 5MTHF (F) is primarily taken up by FRα at the basolateral membrane of the human choroid plexus. The 5MTHF-FRα complex is internalized by receptor-mediated endocytosis, translocated into GPI-anchored protein-enriched early endosomal compartments (GEECs) and further transferred to MVBs. MVBs are late endosomal compartments localized in the endocytic route. A minor proportion of internalized 5MTHF is translocated to PCFT-positive vesicles and transported into the cytoplasma. ILVs of MVBs containing FRα are generated by inward budding of the limiting membrane. These ILVs are released as exosomes into the CSF after fusion of the MVB with the apical cell membrane. Fusion of the limiting membrane of MVBs with the apical membrane explains the presence of FRα molecules on the apical surface of the choroid plexus cells too. FRα-containing exosomes circulate in the CSF, cross the ependymal cell layer and are distributed in the brain parenchyma. FRα-positive exosomes might initially be taken up by astrocytes and from these further delivered to neurons. FRα-negative exosomes hardly cross the ependymal cell layer and are targeted to other brain cells, such as microglia. At higher than normal plasma concentrations of 5MTHF (>100 nM) alternative mechanisms of uptake and transport may provide for transcellular 5MTHF delivery across the choroid plexus. Full size image Our data indicate that human PCFT is localized to intracellular vesicles that are distinct from but may marginally colocalize with FRα-positive ILVs ( Fig. 1d ). Our FRα/PCFT-cotransfection experiments in Z310 choroid plexus cells are consistent with previous reports, demonstrating that PCFT and FRα colocalize to endosomal compartments and that PCFT is responsible for the 5MTHF transport out of acidified endosomal compartments into the cytoplasma [29] , [30] . In case of functional loss of PCFT, the cellular lack of 5MTHF will consequently compromise the function of the choroid plexus and finally also hamper the FRα-dependant 5MTHF export into the CSF. Thus, similar as in the case of KSS, this could explain the fact that patients suffering from hereditary folate malabsorption, the genetic defect of the PCFT, show very low 5MTHF CSF even if they are supplemented with oral folates. Further experimental studies are required to delineate the cooperative functioning of FRα together with the PCFT. PCFT-null mice [31] as well as FRα-deficient mice [32] that can both be rescued by prenatal and/or postnatal folate supplementation provide important tools to substantiate and elaborate the transmembrane transport and the intracellular routing of folates. The unusual cargo transport mechanism of 5MTHF might serve as a stabilizing and buffering system for fluctuations in folate supply and demand of the brain. Most excitingly, our results indicate that exosome targeting into the brain parenchyma crucially depends on the expression of FRα ( Fig. 6 ). Although the molecular mechanism of this selective uptake is presently not clear we hypothesize that FRα induces a signal for exosome internalization. Ependyma cells and astrocytes may function as intermediates for FRα-positive exosomes on their route to other brain cells, such as the neurons. This transport model would explain why normalization of 5MTHF concentration in the CSF does not necessarily correlate with the amelioration of clinical symptoms in patients suffering from a genetic FRα defect. Our investigations provide new insight into the molecular mechanism that might account for cerebral folate transport deficiency and extend this entity to other disorders that affect the choroid plexus, such as the KSS. Although exosomes have been commonly regarded as vehicles for RNA, protein and lipid transfer between cells [33] , [34] , [35] , our studies reveal a novel function of exosome as transport medium for micronutritions. The selective targeting of FRα-expressing exosomes to the brain parenchyma not only substantiate the biological significance of this transport shuttle but also opens up new avenues for therapeutic approaches. By designing their protein expression, exosomes may serve as organ-specific delivery vehicle for therapeutic agents. This strategy has recently been exemplified with exosomes that were engineered to express a neuron-specific peptide derived from the rabies virus [36] . Our work discloses the possibility that targeted manipulation of the choroid plexus or direct application of FRα-positive exosome-like vesicles into the CSF may be a novel strategy to deliver biological active substances into the brain. Using FRα as a natural sorting signal and taking their non-immunogenic properties FRα-positive exosomes represent a particular attractive shuttle system for a broad variety of biomolecules and organic or inorganic compounds. Further scientific exploration of the exosome biology is required to understand their intercellular trafficking and to be able to exploit their full therapeutic potential. Materials Antibodies against the following antigens were used: human FRα (Mov18/ZEL, Alexis Biochemicals, or NCL-L-FRalpha Clone BN3.2, Novocastra), Flot-2 and CD63 (Flot-2, BD Biosciences), transferrin (Dako), ALG-2-interacting protein X (Alix, Covalab), RFC1 (Abcam), GFAP (Dako), ionized calcium-binding adaptor molecule 1 (iba1, WAKO Chemicals), neuron-specific nuclear protein (NeuN, Chemicon) and neurite outgrowth inhibitor protein A (Nogo-A) [37] . An antibody against human PCFT was kindly provided by I. David Goldman (Bronx, New York, USA). Secondary antibodies were purchased from Dianova. FA-FITC was kindly provided by Philip S. Low (West Lafayette, Indiana, USA). PI-PLC from Bacillus cereus was from Sigma. The following inhibitors were used: taurocholate, MTX, p-aminohippuric acid, probenecid, digoxin, brefeldin A and N-ethylmaleimide. All were purchased from Sigma. Human samples All CSF samples were immediately shock-frozen after lumbar puncture and stored at −80 °C. CSF samples recruited from patients suffering from cerebral folate transport deficiency that were recently characterized in detail [9] . CSF samples from nine patients with genetically confirmed KSS were analysed. The KSS patients, six female and three male individuals, were aged between 11 and 25 years at the time of the lumbar puncture. CSF samples from five individuals with suspected hydrocephalus or idiopathic intracranial hypertension, three males and two females that were aged between 2 and 16 years were used as controls. Paraffin sections of human choroid plexus from post-mortem autopsy blocks were retrieved from the Department of Neuropathology, University of Goettingen. Informed consent was obtained from the patients or parents, and the study was approved by the ethical review board of the medical faculty of the University of Goettingen. Cell cultures and transfections Z310 cells were grown in DMEM supplemented with 10% FCS, 10 ng ml −1 epidermal growth factor (Invitrogen) and antibiotics. MDCK cells were maintained MEM supplemented with 10% FCS and antibiotics. The human polarized hepatic cell line HepG2 was grown in RPMI 1640 medium supplemented with 10% FCS and antibiotics. All cells were incubated at 37 °C in 5% CO 2 . Transfections were done using Effectene transfection reagent (Qiagen) and stable transfectants were selected in the presence of the appropriate antibiotics. PCPECs were prepared basically as described previously [38] . Isolated PCPECs were seeded in laminin-coated transwell culture plates (0.4 μm pore size, Costar, Cambridge, MA) with a diameter of 12 mm, using a seeding density of 20 mg wet tissue per cm 2 . At days in vitro 10, the medium was replaced by folate-free RPMI medium (Invitrogen) without serum. The transport experiments were performed on cells at days in vitro 13–15 that exhibited high transepithelial electrical resistance of about 1,000 Ω × cm 2 . Transcytosis assays Transcytosis assays were adapted from Polishchuk et al . [39] Before the experiments, cells were maintained in folate-free RPMI 1640 medium. Filter-grown Z310 or MDCK cells stably expressing FRα incubated on ice for 15 min with 100 nM FA-FITC together with anti-human FRα antibody (Mov18/ZEL) added to the basolateral chamber of the transwell plate. Some filters were fixed immediately after incubation on ice, whereas others were shifted to 37 °C for the indicated time points, fixed and prepared for confocal microscopy. Biochemical evaluation of transcytosis was based on the idea that removal of protein from the basolateral surface will result in decrease of its amount at the apical domain of the plasma membrane [40] . Therefore, filter-grown Z310 or MDCK cells stably expressing FRα were incubated with PI-PLC added to the basolateral medium for the indicated time points. To detect the apical portion of FRα, cells were washed and PI-PLC was added to the apical medium 30 min on ice to collect the receptor from the apical domain of the plasma membrane. Samples were than subjected to western blotting. Exosome preparation Exosomes were prepared from human CSF or from cell culture supernatant by performing sequential centrifugation. Therefore, CSF or supernatant from Z310 cells was centrifuged for 15 min at 1,500 g to remove debris. The supernatant was then subjected to ultracentrifugation at 10,000 g for 45 min and at 100,000 g for 150 min. The collected pellets were finally resuspended in CellLyticM Cell Lysis Reagent (Sigma) and subjected to western blotting. For further analysis, the exosome samples were layered on top of a sucrose gradient and centrifuged for 16 h at 100,000 g . Subsequently, fractions were collected, diluted 1:4 in PBS and centrifuged at 100,000 g for 70 min. Pellets were resuspended in Laemmli sample buffer and subjected to western blotting. For immunofluorescence analysis, the exosome pellet was resuspended in PBS and stained with PKH26 (Sigma). Electron microscopy Exosomes were fixed with 4% paraformaldehyde and absorbed to glow discharged formvar-carbon-coated copper grids. The samples were immunolabelled with antihuman FRα antibody (Mov18/ZEL) or antihuman Flot-2 antibody followed by a rabbit antimouse antibody. The antibodies were detected with Protein A coupled to 10 nm gold particles. After contrasting by neutral uranyl acetate, samples were imaged on a Leo EM912AB-electron microscope (Zeiss) and images were acquired using on axis 2048 × 2048 charge-coupled device camera (Proscan, Schering). Z310 cells were treated with 7 μM monensin for 4 h. Cells were then fixed and prepared for postembedding immunohistochemistry according to ref. 41 . Immunofluorescence microscopy and image analysis Confocal images were acquired on a spinning disk confocal imaging system (UltraView, Perkin-Elmer). The system incorporated an Olympus IX81 inverted microscope using a 100 × 1.4 numerical aperture lens. Excitation wavelengths and filter sets for FITC and Cy3 were as supplied by the manufacturer. Fixed cells labelled with antibodies and/or FA-FITC were optically sectioned into z -stacks. Image processing was performed using the Zeiss LSM image browser software and NIH ImageJ ( http://rsbweb.nih.gov/ij ; Open Source). High-resolution stimulated emission depletion microscopy Exosomes were directly fixed on glass coverslips with 4% paraformaldehyde. Two-colour STED microscopy was performed as previously described [18] , using sheep antimouse polyclonal antibody labelled with Atto590 (for antihuman FRα as first antibody) and goat antirabbit polyclonal antibody conjugated to Atto647N (for Alix as marker for exosomes). The colocalization of FRα and Alix was analysed by using the ‘colocalization threshold’ algorithm from ImageJ. Mass spectrometry analysis Exosomes were prepared as described above and the exosome pellet was directly denatured in Laemmli sample buffer containing 50 mM dithiothreitol for 10 min at 70 °C. Mass spectrometry was then conducted as described previously [42] . Semiquantitative analysis of the relative exosomal protein abundance was determined by the ranking of unweighted spectrum counts with the program Scaffold 3. FRα-mediated 5MTHF uptake and transport analysis For 5MTHF uptake and transport measurements in Z310 cells, 4.2 × 10 4 cells were seeded in laminin-coated transwell culture plates (0.3 cm 2 growth area, 0.4 μm pore size) in folate-free RPMI medium. Seventy-two hours post confluent, cells were loaded with 12.5 or 25 nM [ 3 H]5MTHF in folate-free RPMI medium containing 1% BSA added either to the apical or basolateral chamber of the transwell plates. [3′,5′,7,9- 3 H](6S)-5MTHF was purchased from Moravek Biochemicals (Brea, CA). Cells were then incubated at 37 °C for 1 h and were subsequently washed. Fresh RPMI medium was added containing either 7 μM monensin (Sigma) or 0.5 mg ml −1 rat transferrin (Rockland, Gilbertsville, PA) and cells were then incubated at 37 °C in 5% CO 2 . Samples were removed from the apical and basolateral medium at the indicated time points. To stop the transport experiment, the transwell plates were placed on ice and the cells were washed three times with ice-cold hepes-buffered saline (HBS). Cells were than dissolved in 0.2 M NaOH and protein determination was done with the BCA protein assay (Pierce, Rockford, IL). Radioactivity in medium samples and cell lysates was measured in a liquid scintillation spectrometer. Immunohistochemistry of choroid plexus Immunohistochemistry was carried out as previously described [43] . Staining on human sections was performed using mouse monoclonal FRα antibody (NCL-L-FRalpha) or rabbit polyclonal PCFT antibody followed by horseradish peroxidase-conjugated secondary antibodies. After development, the slides were counterstained with haematoxylin. For immunofluorescence, the sections were treated as described above, except the use of secondary Alexa 488 donkey antimouse or Alexa 546 donkey antirabbit antibodies. Internalization assay Mixed cortical cultures were obtained from neonatal mice and immediately plated on coverslips and incubated in the respective growth medium. Before the internalization assay, exosomes were purified from Z310 cells, stably transfected with FRα or vector and labelled with PKH26 and FA-FITC as described above. The uptake was performed by incubating the cell cultures with exosome dilutions for 2 h at 37 °C and 5% CO 2 . Cells were then fixed, permeabilized and stained with the respective antibodies for immunofluorescence analysis. In vivo experiments were carried out with C57BL/6 mice at the ages between 80 days and 100 days. The mice were anaesthetized with ketamine (100–125 mg kg −1 ) and xylazine (10–12,5 mg ml −1 ) and the intraventricular cannulas were stereotaxically implanted into the lateral ventricle as described previously [44] . Ten microlitres of labelled exosome solution were injected into the intraventricular cannula 4 h before the mice were killed. Intact brains were then dissected, immediately frozen in liquid nitrogen precooled isopentane and stored at −20 °C. For fluorescence analysis, the frozen brain tissues were cryosectioned to a thickness of 10 μm. The frozen sections were fixed in 4% paraformaldehyde for 30 min at room temperature. After washing in PBS, sections were blocked for 1 h in PBS containing 10% (w/v) horse serum and 0.2% BSA. Antibodies against GFAP and NeuN were applied overnight in carrier containing 1% horse serum and 0.2% BSA in PBS. After washing with PBS, slides were incubated with appropriate secondary Alex488 antibodies for 2 h. After washing in PBS, sections were embedded in ProLong Gold with DAPI (4′,6-diamidino-2-phenylindole; Invitrogen). Images were acquired with a confocal microscope (Olympus FV1000). How to cite this article: Grapp, M. et al . Choroid plexus transcytosis and exosome shuttling deliver folate into brain parenchyma. Nat. Commun. 4:2123 doi: 10.1038/ncomms3123 (2013).